Virtual metagenome reconstruction from16S rRNAgene sequences Microbial ecologists have investigated roles of species richness and diversity in a wide variety of ecosystems. Recently, metagenomics have been developed to measure functions in ecosystems, but this approach is cost-intensive. Here we describe a novel method for the rapid and efficient reconstruction of a virtual metagenome in environmental microbial communities without using large-scale genomic sequencing. We demonstrate this approach using 16S rRNA gene sequences obtained from denaturing gradient gel electrophoresis analysis, mapped to fully sequenced genomes, to reconstruct virtual metagenome-like organizations. Furthermore, we validate a virtual metagenome using a published metagenome for cocoa bean fermentation samples, and show that metagenomes reconstructed from biofilm formation samples allow for the study of the gene pool dynamics that are necessary for biofilm growth. Microbial communities have important roles in the bio-cycles of all ecosystems. However, most microbes are uncultivated, and huge metabolic diversities remain to be elucidated. Consequently, with the aim to address and study uncultivated microbes, techniques have been focused on retrieving genes or genomes directly from the environment. To identify species or lineages, conventional techniques employed by microbial ecologists include the use of denaturing gradient gel electrophoresis (DGGE) [1] , [2] to separate 16S rRNA gene sequences from a wide variety of microbes, including uncultivated microbes, obtained directly from the environment [3] . This technique has proven to be applicable in a variety of different environments [4] , [5] , [6] , [7] , [8] , [9] . However, the advent of new-generation sequencers has enabled us to develop new ‘omics’ approaches such as metagenomic analysis using environmental samples. Metagenomic approaches have provided new insights, indicating that species diversity and genetic diversity in an environment underlie microbial ecology [10] , [11] , [12] , [13] , [14] , [15] , [16] . However, metagenomic analysis requires large-scale sequencing data and is still highly cost-intensive. Here, we describe a novel method to reconstruct virtual metagenomes using closely related genomes inferred from completely sequenced genomes based on 16S rRNA gene sequences determined by DGGE analysis. This method is built on the premise that if there is at least one complete genome closely related with a query, the genome can be used as an alternative genome to reconstruct the contents of the query genome. The mixture of such reconstructed genomes in an environmental sample can be regarded as a virtual metagenome. The 16S rRNA gene sequences obtained from the DGGE analysis are mapped to fully sequenced genomes to reconstruct virtual metagenome-like organizations. We validated our method using pyrosequencing metagenome data and the corresponding DGGE experiments, and applied this strategy to the time-course DGGE data in the biofilm reformation experiments. We also demonstrated that the virtual metagenomes reconstructed from the experiments allowed the study of genetic dynamics that occur during biofilm growth. Furthermore, our approach can provide an opportunity to re-evaluate and re-analyse data concerning species richness and diversity from previous experiments in terms of genes. DGGE and homology-based virtual metagenome construction As described above, 16S rRNA gene sequences are commonly sequenced for analysing microbial communities. Using these sequences, our method estimates the phylogeny of query species in the microbial communities. Today, >1,000 genome sequences are publicly available, and these may include enough homologous genomes to predict the query genome contents, although many lineages are not sequenced and their phylogenetic distributions are biased. For this study, 1,137 completely sequenced prokaryotic genomes were obtained from Kyoto Encyclopaedia of Genes and Genomes (KEGG) [17] . We reconstructed a universal phylogenetic tree by using the 16S rRNA genes extracted from the genomes ( Supplementary Fig. S1 ). Our method maps a query 16S rRNA gene sequence to the universal tree, and then identifies closely related genomes ( Fig. 1a and Supplementary Fig. S2 ). The query genome content is predicted by the orthologous gene profile (presence/absence) across the closely related genomes ( Fig. 1a ). KEGG rthology (KO) identifiers are used as a group of orthologous genes. If an orthologous gene exists across multiple closely related genomes, the orthologous gene in the query genome is expressed as a probability defined by the ratio of the closely related genomes having the orthologous genes. In this way, an existence probability for each orthologous gene in the query genome is predicted. 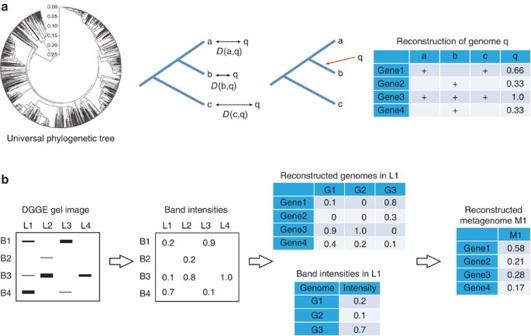Figure 1: Schematic representations of the metagenome reconstruction method. (a) Reconstruction of a genome. The closely related genomes for a query16S rRNAgene sequence are identified from the universal phylogenetic tree. A profile of orthologous genes in the closely related genomes is constructed. The probabilities of the orthologous genes in the query genome are calculated on the basis of the profile. (b) Metagenome reconstruction from DGGE gel image data. The16S rRNAgene was sequenced from the bands. Each genome from the 16S rRNA sequences is reconstructed. In addition, band densities in a gel are transformed into intensity values. A metagenome in a sample is predicted from the reconstructed genomes and their intensities. Figure 1: Schematic representations of the metagenome reconstruction method. ( a ) Reconstruction of a genome. The closely related genomes for a query 16S rRNA gene sequence are identified from the universal phylogenetic tree. A profile of orthologous genes in the closely related genomes is constructed. The probabilities of the orthologous genes in the query genome are calculated on the basis of the profile. ( b ) Metagenome reconstruction from DGGE gel image data. The 16S rRNA gene was sequenced from the bands. Each genome from the 16S rRNA sequences is reconstructed. In addition, band densities in a gel are transformed into intensity values. A metagenome in a sample is predicted from the reconstructed genomes and their intensities. Full size image The scope of our method includes all 16S rRNA genes obtained from biodiversity analyses of microbial communities. In particular, a DGGE analysis of microbial ecology can isolate and identify many 16S rRNA gene sequences and is suitable for the application of our method. A single lane on a DGGE gel can contain multiple different 16S rRNA gene sequences from the same sample. Band densities on a DGGE gel may indicate the relative abundance of organisms in the environment, although there remains some controversy as to the relationship between the band density and the abundance [18] . Assuming that the relative abundance of organisms can be reliably estimated using our method, virtual metagenomes reflecting the abundance of organisms based on band intensities can be reconstructed ( Fig. 1b ), and the functional diversity between the multiple metagenomes reconstructed from different environmental samples used in a DGGE analysis can be compared. However, in this comparison, considering the abundance of DNA applied to the gel, the total value of intensities in a lane on a DGGE gel was normalized to 1.0. In silico validation of virtual metagenome To determine whether a reconstructed genome accurately reflects the query genome, we simulated the reconstruction of KOs in a query genome from completely sequenced genomes. Our results confirmed that when an evolutionary distance (see Methods for the definition) was relatively close, the similarity of content between the closest genomes was also very high ( Fig. 2 ). Consequently, if the closest genome at an evolutionary distance of <0.1 can be identified, the similarity between the query genome and the closest genome may exceed 0.8 ( Fig. 2a ). Furthermore, if the KOs used were limited to those appearing in the KEGG pathways, the similarities showed slightly higher values ( Fig. 2b ). Therefore, if focus is placed on the modules or pathways in functional analysis, our method can reconstruct more reliable genomes/metagenomes. Genome reconstructions using the closely related genomes, including the closest genome, also exhibited high similarities ( Fig. 2c ). Thus, genome reconstructions using our method are effective in cases involving low evolutionary distance thresholds (for example, 0.1), assuming that the genome similarities are sufficiently high. We therefore used 0.1 as the threshold of the evolutionary distance to detect the closest genome from a 16S rRNA sequence. 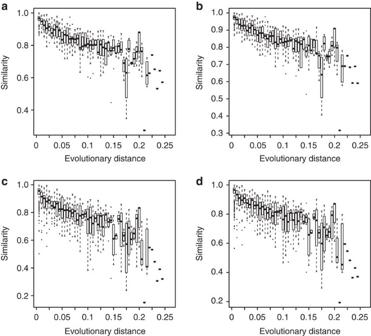Figure 2: Similarity of reconstructed genomes. (a) Genome similarities between the closest genomes are plotted as boxplots and (b) genome similarities between the closest genomes, but the KOs used are limited to those appearing in the KEGG pathways. (c) Genome similarities between a query genome and the genome reconstructed from the query16S rRNAgene and (d) genome similarities between a query genome and the genome reconstructed from the query16S rRNAgene. The KOs used are limited to those appearing in the KEGG pathways. Similarity scores are calculated as a Cosine similarity index. Boxes denote the interquartile range (IQR) between the first and third quartiles and the line inside denotes the median. Whiskers denote the lowest and highest values within 1.5 times IQR from the first and third quartiles, respectively. Circles denote outliers beyond the whiskers. Figure 2: Similarity of reconstructed genomes. ( a ) Genome similarities between the closest genomes are plotted as boxplots and ( b ) genome similarities between the closest genomes, but the KOs used are limited to those appearing in the KEGG pathways. ( c ) Genome similarities between a query genome and the genome reconstructed from the query 16S rRNA gene and ( d ) genome similarities between a query genome and the genome reconstructed from the query 16S rRNA gene. The KOs used are limited to those appearing in the KEGG pathways. Similarity scores are calculated as a Cosine similarity index. Boxes denote the interquartile range (IQR) between the first and third quartiles and the line inside denotes the median. Whiskers denote the lowest and highest values within 1.5 times IQR from the first and third quartiles, respectively. Circles denote outliers beyond the whiskers. Full size image We also validated metagenome reconstructions by extracting 16S rRNA genes from 190 publicly available metagenomes obtained from integrated microbial genomes with microbiome samples [19] . Using these 16S rRNA genes, metagenomes were reconstructed by our method by changing the threshold of an existence probability for a KO that indicates the ratio of closely related genomes possessing the KO to the total number of the closely related genomes. This method was found to be successful, except when the metagenome data did not include 16S rRNA sequences or when mapping of 16S rRNA s were not successful under the evolutionary distance threshold of 0.1. In addition, these 16S rRNA sequences may have included different types of sequences, as they originated from metagenome fragments. However, in this validation, we focused on potential applications of our method for 16S rRNA s from a variety of data sources other than homogenous sequences obtained from DGGE or similar techniques. The similarity between a query metagenome and the reconstructed metagenome was correlated with the number of unique KO species, particularly when we used all KO species included in the closely related genomes (existence probability threshold: 0.0) ( Fig. 3a ). Some metagenomic samples in Fig. 3a exhibited >0.8 similarity ( Supplementary Table S1 ). However, the use of higher thresholds of existence probabilities resulted in low similarities in the metagenome samples possessing large numbers of KO species ( Fig. 3b–f ), which suggests that species-specific genes included in the closely related genomes are also important for reconstruction of metagenomes. 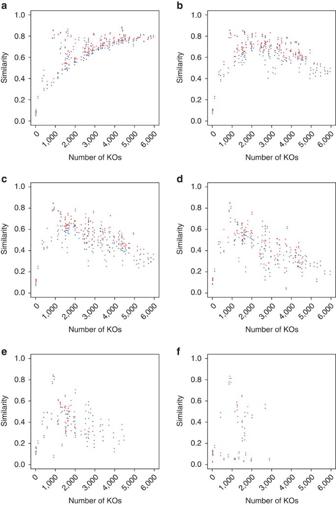Figure 3: Similarity of reconstructed metagenomes. Metagenomic similarities between a query metagenome and the reconstructed metagenome from the query16S rRNAgenes with the thresholds of the existence probabilities (a) 0.0, (b) 0.2, (c) 0.4, (d) 0.6, (e) 0.8 and (f) 1.0. Blue indicates the similarities based on all KOs, and red, based on the KOs appearing in the KEGG pathways. Thexaxis indicates the number of unique KOs in each reconstructed metagenome. Figure 3: Similarity of reconstructed metagenomes. Metagenomic similarities between a query metagenome and the reconstructed metagenome from the query 16S rRNA genes with the thresholds of the existence probabilities ( a ) 0.0, ( b ) 0.2, ( c ) 0.4, ( d ) 0.6, ( e ) 0.8 and ( f ) 1.0. Blue indicates the similarities based on all KOs, and red, based on the KOs appearing in the KEGG pathways. The x axis indicates the number of unique KOs in each reconstructed metagenome. Full size image Comparison with a metagenome assembled from sequencing Recently, Papalexandratou et al . [20] published a metagenome analysis of cocoa bean fermentation samples determined by pyrosequencing technique. A DGGE analysis of the same samples was also previously performed by the same group [21] . We therefore compared the virtual metagenome reconstructed by our method and the real metagenome from the same cocoa bean fermentation samples. The comparison of KO content between the two sets indicated a high similarity at low existence probabilities ( Fig. 4a ). The highest genome similarity calculated was 0.78 with an existence probability of 0.08. It was surprising to observe that the virtual metagenome reflected the real metagenome at ~0.8 similarity. At existence probabilities >0.1, the genome similarities decreased drastically. This suggests that rare genes conserved in part of the closely related genomes would be quite important for reconstructing the metagenome from 16S rRNA sequences. In addition, comparison of KEGG BRITE functional categories for these two metagenomes showed similar distribution (Pearson’s correlation coefficient: 0.9624, P <0.0001) ( Fig. 4b ). Furthermore, similar distributions were observed between the two metagenomes by using more granular functional categories (Pearson’s correlation coefficient: 0.8083, P <0.0001) ( Supplementary Fig. S3 ). Therefore, a virtual metagenome reconstructed by our method could be also expected to reflect functions of a real metagenome. 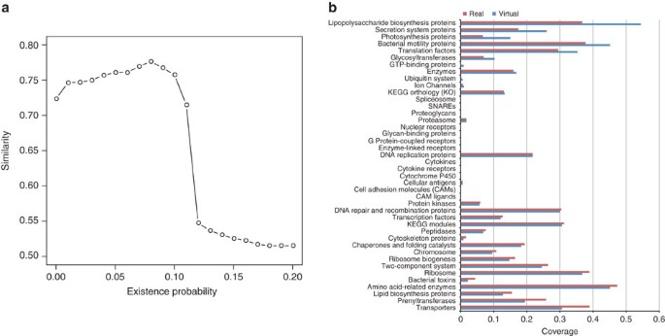Figure 4: Comparison between virtual and real metagenomes from cocoa fermentation samples. (a) Similarity of virtual metagenomes reconstructed from DGGE data obtained from cocoa fermentation samples. Genome similarities for each threshold of probabilities, where orthologous genes were conserved in the closely related genomes, are plotted. Similarity scores are calculated as a Cosine similarity index. (b) Functional distributions between virtual and real metagenomes. KEGG BRITE categories at the first hierarchical level were counted in the virtual and real metagenomes. Thexaxis indicates coverage of KOs in each category. Figure 4: Comparison between virtual and real metagenomes from cocoa fermentation samples. ( a ) Similarity of virtual metagenomes reconstructed from DGGE data obtained from cocoa fermentation samples. Genome similarities for each threshold of probabilities, where orthologous genes were conserved in the closely related genomes, are plotted. Similarity scores are calculated as a Cosine similarity index. ( b ) Functional distributions between virtual and real metagenomes. KEGG BRITE categories at the first hierarchical level were counted in the virtual and real metagenomes. The x axis indicates coverage of KOs in each category. Full size image Application to biofilm reformation To apply our method to the 16S rRNA sequences obtained from biofilm formation samples, we sequenced 16S rRNA genes obtained from the DGGE analysis of the biofilm formation processes previously reported [22] . After the removal of the biofilms from the surface of reeds inhabiting Lake Biwa in Japan, the process of reformation of the biofilm on the surface was measured by DGGE experiments performed from 19 May 2008 to 23 July 2008 ( Supplementary Table S2 ). Data samplings were acquired beginning on two different days, with the samples identified as FP1 and FP2, whereas the sample acquired from the lake water as a control was identified as LW. The suffix in sample names indicates the number of days elapsed from the start of the experiment. The authors reported that the microbial communities were different between the biofilm and the lake water surrounding it, and also between the experimental periods. Subsequently, we applied our method to this data set and reconstructed metagenomes from the time-course data related to the biofilm reformation process. To observe functions specific to each sample, we mapped modules obtained from KEGG MODULE and KEGG BRITE functional categories. Subsequently, we performed clustering of the module ( Fig. 5a and Supplementary Fig. S4 ) and category ( Fig. 5c and Supplementary Fig. S5 ) profiles to analyse the time-course dynamics of gene pools in the environments. 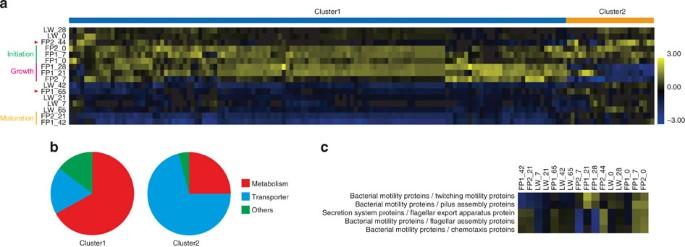Figure 5: Functional transitions through biofilm formation. (a) Clustering of a functional module profile. Module enrichments are colour coded. Clustering of module transition patterns provides two clusters (cluster 1 is blue and cluster 2 is orange). The prefix FP1 in the sample name indicates the early experiments, whereas FP2 indicates the later experiments. LW indicates the data obtained from the lake water. The numeric suffix in the sample names indicates the number of days elapsed after the experiment started. The stages of biofilm formation are described on the left side of the sample names. Red arrows indicate the final stage. (b) Pie charts of functions in clusters 1 and 2. Red indicates transporter-related modules, blue indicates metabolism-related modules and green indicates other functions. (c) Clustering of a functional category profile related to motility and flagella. Colour densities are the same as ina. Figure 5: Functional transitions through biofilm formation. ( a ) Clustering of a functional module profile. Module enrichments are colour coded. Clustering of module transition patterns provides two clusters (cluster 1 is blue and cluster 2 is orange). The prefix FP1 in the sample name indicates the early experiments, whereas FP2 indicates the later experiments. LW indicates the data obtained from the lake water. The numeric suffix in the sample names indicates the number of days elapsed after the experiment started. The stages of biofilm formation are described on the left side of the sample names. Red arrows indicate the final stage. ( b ) Pie charts of functions in clusters 1 and 2. Red indicates transporter-related modules, blue indicates metabolism-related modules and green indicates other functions. ( c ) Clustering of a functional category profile related to motility and flagella. Colour densities are the same as in a . Full size image Monitoring transitions in biofilm formation The pattern of module enrichment was separated into two large clusters (clusters 1 and 2). Cluster 1, in which metabolism-related modules were enriched ( P =0.0072, two-tailed Fisher’s exact test), was dominant in the initiation and growth stages in biofilm formation, whereas cluster 2, in which transporter-related modules were enriched ( P =0.0067, two-tailed Fisher’s exact test), was dominant in the initiation and maturation stages ( Fig. 5a ). In the initiation stage of biofilm formation, transporter- and biosynthesis-related modules were enriched. Biosynthesis-related modules were then enriched in the growth stage of the biofilms, resulting in the relative decrease of transporters. Finally, during the maturation stage of the biofilms, biosynthesis-related modules were no longer dominant, but the transporters that had relatively decreased in the growth stage were again enriched. In addition, flagellar/chemotaxis-related functional categories appeared during the initiation and maturation stages, and subsequently relatively decreased during the growth stage ( Fig. 5c ). In the biofilm formation model, bacterial cells attach reversibly to the surface [23] , [24] , [25] , [26] , [27] . The cells then produce exopolymeric substances such as lipopolysaccharides and lose the flagella-driven motility. After the biofilm development reaches the maturation stage, motile cells are dispersed from the microcolonies [26] . In addition, during the biofilm growth stage involving the production of exopolysaccharides, flagella synthesis was observed to decrease presumably because flagella may destabilize the structure of biofilms [27] . Therefore, the results of previous studies of biofilm formation [23] , [24] , [25] , [26] , [27] were consistent with the gene pool dynamics we observed in this study. Although FP2 began 3 weeks after FP1, FP2 exhibited rapid growth and reached the maturation stage at almost the same time as FP1, possibly due to environmental conditions such as temperature. The clustering of the experiment periods accurately grouped the samples at the same stages into the same clusters ( Fig. 5a and Supplementary Fig. S6 ). These results indicate that the transition pattern of functional modules could reflect the order of the biofilm growth ( Fig. 5a and Supplementary Fig. S4 ). Furthermore, this finding is consistent with results reported by Hiraki et al . [22] that the order of phenotypic transitions (that is, the physical appearance of the biofilm, wet-weight, nutrient ion concentrations, bacterial density, and EPS characteristics in the biofilm) during biofilm formation was the same in two different experimental periods. The final stage of biofilm formation (FP1_65 and FP2_44) revealed two different patterns of functions, where FP1_65 was similar to the maturation stage, whereas FP2_44 was similar to the initiation stage, although both samples most closely resembled the lake water samples. Because biofilm is destroyed in the final stage, it was assumed that the functions at this stage were quite unstable. Our approach to reconstruction of metagenomes, without reliance on large-scale sequencing, is a strong tool to observe the dynamics of genes in a variety of environments. One of the reasons that we were able to successfully reconstruct virtual metagenomes and observe their functional properties, is that both fermentation and biofilms may comprise closed systems that are limited in terms of species and genetic diversity, thus allowing us to predict the proper, closely related genomes from only 16S rRNA s. Our results, indicating that the virtual metagenomes reflect real functional compositions and actual transitions of gene pools even though they were virtually reconstructed from DGGE, suggest that our method is sufficiently effective and useful for this type of research. In addition, this technique will have a great impact in the medical field because it applies to human gut microbiota, clinical monitoring in real-life settings, or the use of biofilms in medical devices. Although our method is not readily applicable in cases where the most closely related genomes are unmapped, future efforts to increase the breadth and availability of completely sequenced genomes will compensate for this problem. In summary, we demonstrated and validated a rapid and efficient reconstruction strategy for analysing genomes/metagenomes from 16S rRNA genes without using large-scale sequencing, and successfully evaluated genetic dynamics in actual environmental samples. Our approach provides an opportunity to re-evaluate massive volumes of information on species diversity by using 16S rRNA gene sequence data accumulated in previous experiments performed by microbial ecologists, and to re-analyse these data in terms of genes/genomes to provide deeper insights into the microbial functions in such environments. Construction of the universal phylogenetic tree In total, 1,137 prokaryotic genomes were downloaded from KEGG [17] in June 2011. We collected a reference RNA set of 16S rRNA gene sequences, selecting a representative sequence from each genome if it included multiple 16S rRNA genes. Subsequently, we computed the multiple sequence alignment for the reference sequence with MAFFT [28] and constructed the phylogenetic tree with MEGA [29] by using the neighbor-joining method and the maximum composite likelihood model. Mapping of 16S rRNA sequences to the universal tree We mapped the query sequence by comparing the distances between a query and the reference RNA set on the universal tree. Evolutionary distances between a query 16S rRNA gene sequence against the reference RNA set were computed with the closest 16S rRNA sequence in the reference RNA set selected as an initial sequence. In these calculations, q is the query sequence, t is a leaf or an internal node on the path from the initial sequence to the root on the universal tree and s is the sibling node of t (see Supplementary Fig. S2 ). Along with the path from the initial sequence to the root, we computed the distances between q , t and s, and mapped the query as a sister clade of t, where the distances could be described with the following inequality (1): where D ( t , s ) and D ( t , q ) are distances between t and s and between t and q , respectively. Here a distance between two nodes is computed using the following equation (2): where X ( Y ) is the set of all descendant sequences of node x ( y ), and d ( x i , y j ) is the evolutionary distance between x i and y j . Evolutionary distances were calculated with PHYLIP [30] using the default parameters. All of the evolutionary distances used in this study were based on 16S rRNA sequences, obtained from complete genomes, DGGE analyses and metagenome data. Reconstruction of a genome The query genome was predicted by the closely related genomes, including the closest one determined by the above mapping process. KOs in all closely related genomes were extracted, and a profile of the presence or absence across the genomes was determined. On the basis of the profile, the existence probability E kq for a particular KO ( k ) in a query genome ( q ) was defined by the ratio of the number of closely related genomes possessing the KO to the total number of the closely related genomes. In cases where it was difficult to identify the closest genome from multiple genomes that were indistinguishable based on evolutionary distances, we used all the closest genomes and the closely related genomes to calculate the probability. In this way, the functional content of the genome was expressed as a vector of existence probabilities of KOs. Determination of 16S rRNA sequences in biofilm formation We sequenced the 16S rRNA genes obtained from the DGGE analysis reported in a previous study [22] . We then excised most of the visible DGGE bands (112 of 155) from a gel with a sterilized 1.0-ml pipette tip and suspended them in sterilized Tris-EDTA buffer (10 mM Tris–HCl, 1 mM EDTA, adjusted to pH 8.0). DNA was recovered from the gels by freezing and subsequent thawing. The recovered DNA (77 of 112) was amplified using a primer set for bacteria: 341f-GC ( Escherichia coli position 341–357), 5′- CGCCCGCCGCGCCCCGCGCCCGTCCCGCCGCCCCCGCCCG CCTACGGGAGGCAGCAG-3′ (underlined sequence denotes the GC clamp) and 907r ( E. coli position 926–907), 5′-CCCCGTCAATTCATTTGAGTTT-3′. The amplification conditions were as follows: 95 °C for 3 min (initial denaturation), followed by 30 cycles of 95 °C for 1 min, 52 °C for 1 min and 72 °C for 2 min, with a final extension step of 72 °C for 10 min. The recovered DNA (77 of 112) was then amplified and the mobility was checked on DGGE gels under the same conditions reported in the previous DGGE study [22] . The DNA, which could be amplified and whose mobility could be confirmed, was then sequenced by Fasmac DNA Sequence Service (Kanagawa, Japan). The phylogenetic analysis was conducted using ca. 500 bp. All determined sequences of 16S rRNA genes have been submitted to the DDBJ under the accession numbers ( Supplementary Table S3 ). Band intensity in a DGGE gel image A DGGE gel image was processed using a banding pattern image analyser (TL120; Nonlinear Dynamics Ltd., Newcastle upon Tyne, UK), and each band density in the gel was transformed into an intensity value ( Supplementary Tables S4–S7 ). Because the DNA abundance applied into each lane in the gel could differ, the intensity value was normalized by the total intensity in a lane. The intensity for the query genome q was defined by equation (3): where B q denotes band intensity corresponding to query q , and L q denotes a set of intensities for bands in the lane where the query band exists. Reconstruction of a metagenome Each band in the DGGE gel corresponds to a 16S rRNA gene sequence. In other words, a genome reconstructed from the sequence correspond to the relative abundance of band intensity in a sample. Although there were some unidentified bands, the remaining 16S rRNA sequences located on the same rows were used as alternatives because a band at the same row position was assumed to represent the same 16S rRNA sequence. If multiple different 16S rRNA sequences were identified in the different lanes in the same row, an unidentified band in the row was presumed, as the identified sequences exist equally in the band. When 16S rRNAs of all the bands in the same row were unidentified because of low densities, we rejected them. Finally, the existence probabilities of orthologous genes in the reconstructed genome were transformed into relative existence probabilities by multiplying the normalized band intensity. The relative existence probability of a KO k , R kq for the query genome q was defined by following equation (4): where E kq denotes the existence probability defined above. Finally, the relative existence probability of a KO in a reconstructed metagenome was defined by equation (5): where G l denotes a set of genomes on the lane l . Reconstruction of biological functions We downloaded and utilized information for a total of 371 biological modules from KEGG MODULE. Each module is described by a combination of KO identifiers, and some modules include possible multiple combinations that function biologically in an organism. Therefore, we first extracted the functionally meaningful combinations of KOs in a module. The average of the relative existence probabilities in the KO combination was calculated, and the maximum value of the averages in a module was assigned to the module for the clustering analysis. We also downloaded KEGG BRITE, the hierarchical classifications of KOs. The categories from each hierarchy level were extracted, and the average for the relative existence probabilities of KOs included in a category was calculated for the clustering analysis. Clustering of functional profiles The DGGE gel image that was used included 16 different samples. Therefore, each module or category was expressed as a vector including 16 values. In both the modules and categories, we discarded a vector with all values <0.3. To compare patterns of the abundance of the modules or changes in categories throughout biofilm formation, the values in a vector were transformed into z -scores. Subsequently, the vectors of the modules and categories were clustered using the Euclidean distance and Ward’s method by the R package statistical software ( http://www.r-project.org/ ). Validation for reconstruction of genomes We calculated genomic similarity between a query genome and the closest genome in the KEGG genomes without the query genome. The similarity was evaluated as a Cosine similarity based on profiles for orthologous genes (KOs) between them. Furthermore, the similarities between a query genome and the genome reconstructed from the query 16S rRNA sequence, with all genes included in the closely related genomes, were calculated. In addition, in both cases, the similarity was calculated when the KOs used were limited to those appearing in the KEGG pathways. Validation for reconstruction of metagenomes We downloaded 190 metagenomes from integrated microbial genomes with microbiome sample [19] in June 2011 ( Supplementary Table S1 ). The 16S rRNA genes were extracted by the original annotations from the metagenome data and applied to our genome reconstruction method, normalized by the number of 16S rRNA genes in a sample. In each metagenome sample, the reconstructed genomes from 16S rRNA sequences obtained from the sample were equally combined into a metagenome-like data set. To evaluate the accuracy of the reconstruction, Cosine similarity of KOs between the reconstructed genome and the original metagenome was calculated. Validation with a real metagenome We downloaded metagenome data of the cocoa bean fermentation samples [21] from NCBI SRA ( http://www.ncbi.nlm.nih.gov/sra/ ). We assembled the reads using Celera Assembler version 7.0 ( http://www.jcvi.org/cms/research/projects/cabog/ ) with the default parameters. Genes were predicted by MetaGene [31] with a multiple species option. We used the KEGG KAAS algorithm [32] against the genome data sets to assign KO identifiers to the genes. In addition, we obtained 16S rRNA gene sequences from DGGE in the same cocoa bean fermentation samples [19] . We applied these 16S rRNA sequences to our virtual metagenome reconstruction method. We compared the KOs shared between the real and virtual metagenomes to calculate Cosine similarity. Finally, we calculated coverage of KOs in a KEGG BRITE category at the first-level hierarchy and at the third level as a granular level. Statistics Correlations of distributions between functional category profiles in the virtual and real metagenomes were computed, based on Pearson’s correlation coefficients [11] . Significant modules in the clustering analysis were identified using Fisher’s exact test [11] . Correction for multiple testing for Fisher’s exact test was performed based on the Benjamini–Hochberg False Discovery Rate (corrected P -value<0.05). Accession codes: All 16S rRNA sequences have been deposited in the DDBJ database under the accession codes AB697766 to AB697824 . How to cite this article: Okuda, S. et al . Virtual metagenome reconstruction from 16S rRNA gene sequences. Nat. Commun. 3:1203 doi: 10.1038/ncomms2203 (2012).